The use of the sex pheromone as an evolutionary solution to food source selection in caterpillars Sex pheromones are released by adults of a species to elicit a sexual interaction with the other sex of the same species. Here we report an unexpected effect of a moth sex pheromone on the caterpillars of the same species. We demonstrate that larvae of the cotton leafworm Spodoptera littoralis are attracted by the moth sex pheromone and that this phenomenon is independent of sex determination. In addition, we show that the olfactory sensilla carried by the caterpillar antennae are sensitive to the pheromone and that the caterpillar sensilla express pheromone-binding proteins that are used by adult antennae to bind pheromone components. Finally, we demonstrate that the larvae are preferentially attracted to a food source when it contains the sex pheromone main component. A possible interpretation of these results is that the sex pheromone is used to promote food search in caterpillars, opening potential new routes for insect pest management. Through metamorphosis, holometabolous insects split their life cycle into markedly different forms with radically different physiologies and ecologies. In Lepidoptera, the larval form consists of caterpillars that feed, grow and accumulate energy, whereas the adults assume the reproductive responsibilities and species dispersal. The behaviours of the larvae and the adults, such as searching for a food source (moth, caterpillar) or an appropriate oviposition site (female) or a mate (male), are largely ruled by olfaction. However, the olfactory organs of the adult and larval stages are morphologically different. Although the adults have a pair of large antennae covered with tens of thousands of olfactory sensilla, caterpillars possess two principal organs: a pair of antennae and a pair of maxillary palps [1] , [2] , each of which equipped with a reduced number of olfactory sensilla. Each caterpillar antenna has only three olfactory sensilla; two are located on the second antennal segment and one is located on the third segment [2] , [3] , [4] . The maxillary palps bear eight sensilla [5] . Together, the larval antennae and palps house 78 olfactory receptor neurons (ORNs) [1] , 16 of which are located in the antenna [1] , [3] . In turn, the adult antennae bear thousands of olfactory sensilla, each housing two or three ORNs [6] . Accordingly, adults and larvae express different, although somewhat overlapping, olfactory receptor (OR) repertoires in their ORNs. The silkworm Bombyx mori larvae, for instance, express a total of 24 ORs, 18 of which are shared by the adults, which express 35 ORs [7] . Adult male antennae are highly specialized in the detection of the sex pheromone emitted by females [8] . Correspondingly, their antennae express sex pheromone receptors (PRs) and pheromone-binding proteins (PBPs), the latter being thought to solubilize pheromone molecules and transport them through the sensillar lymph to the PRs [9] . Both the PRs and the PBPs have been reported to be exclusively expressed in adults [2] , [4] , [7] , [10] , [11] . These ecological and molecular data suggest that the detection of sex pheromones is restricted to the adult stage. However, intriguing molecular clues have caused us to reevaluate this paradigm. First, PBP expression has been recently illustrated in the larval heads of B. mori [12] , although at a low level. Second, a larval OR that responds to bombykol, the sex pheromone of this species, has been identified [7] . These observations suggest that the adult sex pheromone might be a relevant, although unexpected, olfactory cue for caterpillars. In this study, using behavioural, electrophysiological and molecular data accumulated for the noctuid moth Spodoptera littoralis , we provide evidence that caterpillars can detect and are attracted to the adult sex pheromone. First, we show that S. littoralis larvae walk dose-dependently towards a sex pheromone source, but that they do not respond to a heterospecific sex pheromone. Second, we show that the larval antennae house ORNs responding to the sex pheromone. Third, we found that the larval antennae express the three PBPs previously identified in adults. Finally, we found, using a choice test, that the larvae are more attracted to a food source containing the main sex pheromone component than to food that does not contain it. Thus, we demonstrate that the larvae can detect and orient themselves towards an adult-specific sex signal, and we propose that caterpillars use this unexpected cue to enhance food detection. Behavioural responses of larvae to a sex pheromone source We used a servosphere assay to examine the chemotaxis response ( Fig. 1a ) of S. littoralis L3-L4 larvae to different stimuli: hexanol, which has previously been reported to induce an attractive behaviour in caterpillars [13] , S. littoralis sex pheromone gland extracts (SlitPGE), synthetic Z9,E11-14:Ac (the main S. littoralis sex pheromone component) [14] and sex PGEs from the cabbage armyworm Mamestra brassicae (MbraPGE). 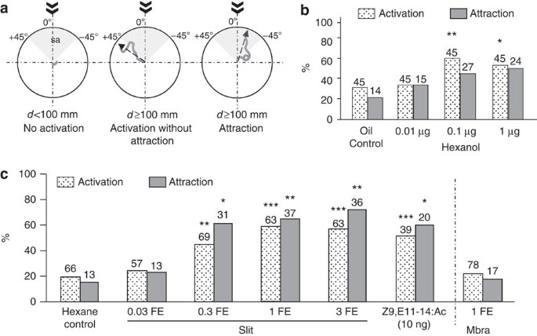Figure 1: Behavioural responses ofS. littoralisL3-L4 larvae to volatile compounds. (a) The circles illustrate the three types of paths (characteristic paths represented here) defined according to the path length (d) and the path position with respect to the odour source (the source area (sa) is the upstream quadrant centered along the air-flow axis). According to our criteria, the three types of paths correspond to: no activation (d<100 mm) (left), activation without attraction (d≥ 100 mm, but the mean angle of the path is out of the sa) (middle) and attraction (d≥ 100 mm, and the mean angle of the path is within the sa) (right). Arrows on the tops of circles indicate the odour source position and the air-flow direction. The arrows within circles indicate the mean vector of the path. (b) Percentages of activated and attracted larvae exposed to paraffin oil (control) and three doses of hexanol. (c) Percentages of activated and attracted larvae exposed to hexane (control), four doses of SlitPGE, 10 ng of Z9,E11-14:Ac and 1 FE of MbraPGE. Significant differences compared with the control are indicated by *P<0.05, **P<0.01 or ***P<0.001, respectively; logistic regression. The total numbers of tested larvae and of activated larvae cap the % activation and % attraction bars, respectively. Figure 1: Behavioural responses of S. littoralis L3-L4 larvae to volatile compounds. ( a ) The circles illustrate the three types of paths (characteristic paths represented here) defined according to the path length ( d ) and the path position with respect to the odour source (the source area (sa) is the upstream quadrant centered along the air-flow axis). According to our criteria, the three types of paths correspond to: no activation ( d <100 mm) (left), activation without attraction ( d ≥ 100 mm, but the mean angle of the path is out of the sa) (middle) and attraction ( d ≥ 100 mm, and the mean angle of the path is within the sa) (right). Arrows on the tops of circles indicate the odour source position and the air-flow direction. The arrows within circles indicate the mean vector of the path. ( b ) Percentages of activated and attracted larvae exposed to paraffin oil (control) and three doses of hexanol. ( c ) Percentages of activated and attracted larvae exposed to hexane (control), four doses of SlitPGE, 10 ng of Z9,E11-14:Ac and 1 FE of MbraPGE. Significant differences compared with the control are indicated by * P <0.05, ** P <0.01 or *** P <0.001, respectively; logistic regression. The total numbers of tested larvae and of activated larvae cap the % activation and % attraction bars, respectively. Full size image Activation and attraction behaviours were defined according to the path length (at least 100 mm) and the angle of the mean vector of the path with the source (less than 45°) (Methods) ( Fig. 1a ). Hexanol triggered significant activation at 0.1 and 1 μg (logistic regression, z =−2.71, P =0.007) ( Fig. 1b ), and a weak attraction, although not statistically significant, was observed ( G =3.671; df=3; P =0.30). Surprisingly, the larvae showed activation in response to SlitPGE at doses starting at 0.3 female equivalent (FE) ( z =−3.06, P =0.002), with a maximum of 59% of activated larvae at 1 FE ( z =−4.38, P =0.001), and attraction was also found from 0.3 (61%; z =−2.54, P =0.011) to 3 FE (72%; z =−3.11, P =0.002) ( Fig. 1c ). Similarly, Z9,E11-14:Ac caused significant activation and attraction starting at 10 ng (corresponding to 2 FE) (60% of the attracted larvae; z =−2.36, P =0.018) ( Fig. 1c ). Neither activation nor attraction was observed in the larvae challenged with 1 FE of MbraPGE. Next, we examined whether the antennae, the maxillary palps or both were involved in sex pheromone detection. We inhibited olfactory detection from the antennae by covering them with low-melting-point wax. The sham control animals exhibited both activation and attraction similar to those of the non-treated animals at 1 FE of SlitPGE; however, the larvae with wax-embedded antennae were not activated and thus not attracted ( Fig. 2 ). 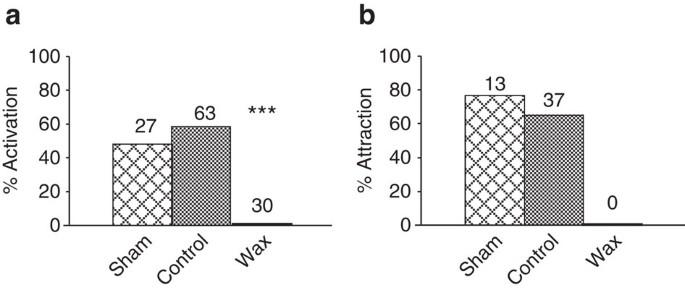Figure 2: Effect of wax-embeddingS. littoralislarvae antennae. Activation (a) and attraction (b) percentages of L3-L4 larvae with intact antennae (control), wax-embedded antennae (wax) and sham controls (sham) exposed to an air-flow enriched with SlitPGE (1 FE). No difference was observed between the intact and sham control larvae (z=0.92,P>0.35; logistic regression), whereas antennae-blocked larvae were neither activated nor attracted. Significant differences compared with the control are indicated by ***P<0.001 (logistic regression). The total numbers of tested larvae and of activated larvae cap the % activation and % attraction bars, respectively. Figure 2: Effect of wax-embedding S. littoralis larvae antennae. Activation ( a ) and attraction ( b ) percentages of L3-L4 larvae with intact antennae (control), wax-embedded antennae (wax) and sham controls (sham) exposed to an air-flow enriched with SlitPGE (1 FE). No difference was observed between the intact and sham control larvae ( z =0.92, P >0.35; logistic regression), whereas antennae-blocked larvae were neither activated nor attracted. Significant differences compared with the control are indicated by *** P <0.001 (logistic regression). The total numbers of tested larvae and of activated larvae cap the % activation and % attraction bars, respectively. Full size image Sex status and larval stage effects To determine whether the attraction towards a sex pheromone source depended on the larval instar, we replicated the experiments with L1-L2 larvae. No significant differences were observed in either the activation or the attraction responses between L1-L2 and L3-L4 exposed to 1 FE of SlitPGE ( Supplementary Fig. S1 ). Next, we investigated whether the larvae responded differently to the sex pheromone signal according to the sex information carried by the larvae. The percentages of activation and attraction were compared in caterpillars that transformed into males and females, respectively. No sex effect was observed for either response parameter, regardless of the SlitPGE dose used ( Supplementary Fig. S2 ). Effect of pheromone on caterpillar food choice When given a choice between a regular diet and a diet plus Z9,E11-14:Ac (10 ng), the larvae showed a preferential attraction towards the diet plus Z9,E11-14:Ac, with positive choice indexes (preference) that were significantly different from 0 (0=no preference) at 4, 6, 10, 14, 20 and 30 min ( Fig. 3a,b ). When larvae were challenged with two spots of regular diet, the calculated choice indexes were not different from 0 at any time. 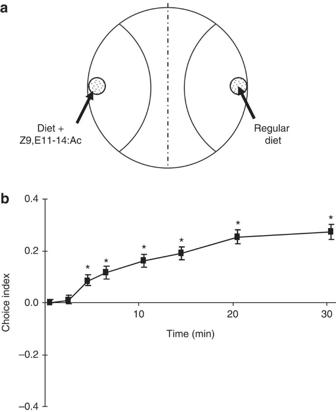Figure 3: Effect of pheromone on food choice. (a) Choice test design. Two areas are defined by arc circles centered one on the regular diet spot and one on the diet+pheromone spot (radius 5.5 cm). (b) Choice index (± s.e.m.) to sex pheromone (10 ng of Z9,E11-14:Ac)+food (1 g diet) at different time points (0–30 min) (20 boxes per point, 8–10 larvae per box). Choice indexes significantly different from 0 are indicated by * (4 min:P=0.042; 6 min:P=0.022; 10 min:P=0.008; 14 min:P=0.003; 20 min:P=0.001; 30 min:P=0.001; Mood test). No difference with 0 was observed at any time point for the choice index in the control experiment (1 g regular diet versus 1 g regular diet). Figure 3: Effect of pheromone on food choice. ( a ) Choice test design. Two areas are defined by arc circles centered one on the regular diet spot and one on the diet+pheromone spot (radius 5.5 cm). ( b ) Choice index (± s.e.m.) to sex pheromone (10 ng of Z9,E11-14:Ac)+food (1 g diet) at different time points (0–30 min) (20 boxes per point, 8–10 larvae per box). Choice indexes significantly different from 0 are indicated by * (4 min: P =0.042; 6 min: P =0.022; 10 min: P =0.008; 14 min: P =0.003; 20 min: P =0.001; 30 min: P =0.001; Mood test). No difference with 0 was observed at any time point for the choice index in the control experiment (1 g regular diet versus 1 g regular diet). Full size image Electrophysiological response of larvae antennae to a pheromone source S. littoralis larval antennae, typical of Lepidoptera, consist of three segments ( Fig. 4a ). All electrophysiological recordings were obtained from one of the two olfactory sensilla located on segment II ( Fig. 4b ). Given the high level of spontaneous activity, we were not able to separate the activity of the different neurons (usually four) housed in the sensillum; therefore, the global firing activity was measured. The firing activities upon the PGE or Z9,E11-14:Ac stimulation were significantly higher than those upon hexane stimulation for all doses (Mann–Whitney, P <0.001) ( Fig. 4c and 4d ). The firing activities increased upon stimulation with increasing doses of SlitPGE (ANOVA, F test, slope 47.6±4.7, P= 0.0001), MbraPGE (slope 27.7±4.7, P= 0.0001) or Z9,E11-14:Ac (slope 0.09±0.01, P= 0.0001). The highest firing rates were obtained upon stimulation with 2 FE of SlitPGE, and a decrease was observed at 3 FE, possibly due to ORN adaptation at a high dosage. For comparison, 1 FE of SlitPGE generated 145.4±13.6 spikes s −1 (average±s.e.m.) above the background firing level, whereas 1 FE of MbraPGE generated 78.4±17.4 spikes s −1 and 5 ng of Z9,E11-14:Ac (amount detected in 1 FE of gland extract) triggered 82.4±8.9 spikes s −1 ( Supplementary Fig. S3 ). 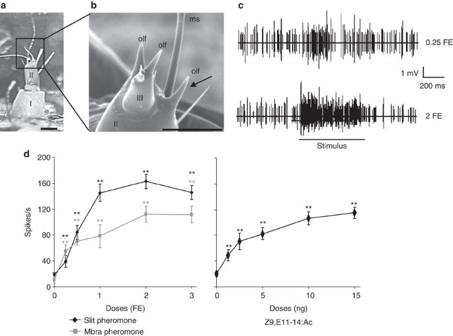Figure 4: Single sensillum recordings from olfactory sensilla located on larval antennae. (a) General view of the antenna of aS. littoralislarva, showing two of the three antennal segments (I and II). Bar: 500 μm. (b) Magnified scanning electron microscopy view of the third antennal segment (III): olf, olfactory sensilla; ms, mechanosensory sensillum; arrow, the sensillum used for electrophysiological recordings. Bar: 50 μm. (c) Representative traces of single sensillum recordings from antennal sensilla showing responses to the SlitPGE. (d) Electrophysiological responses to different doses of SlitPGE and MbraPGE, and synthetic Z9,E11-14:Ac. The action potentials were generated by at least three ORNs. Each data point represents the mean (±s.e.m.) firing rate, which was calculated as described in the Methods section (n=8–12 larvae, one stimulation per larva). Significant differences compared with the control (hexane, data point 0) are indicated by ** (Mann–Whitney,P<0.001). Figure 4: Single sensillum recordings from olfactory sensilla located on larval antennae. ( a ) General view of the antenna of a S. littoralis larva, showing two of the three antennal segments (I and II). Bar: 500 μm. ( b ) Magnified scanning electron microscopy view of the third antennal segment (III): olf, olfactory sensilla; ms, mechanosensory sensillum; arrow, the sensillum used for electrophysiological recordings. Bar: 50 μm. ( c ) Representative traces of single sensillum recordings from antennal sensilla showing responses to the SlitPGE. ( d ) Electrophysiological responses to different doses of SlitPGE and MbraPGE, and synthetic Z9,E11-14:Ac. The action potentials were generated by at least three ORNs. Each data point represents the mean (±s.e.m.) firing rate, which was calculated as described in the Methods section ( n =8–12 larvae, one stimulation per larva). Significant differences compared with the control (hexane, data point 0) are indicated by ** (Mann–Whitney, P <0.001). Full size image Expression of PBPs in larval antennae We then investigated whether caterpillars express the genes identified in the adult antennae that are thought to be involved in sex pheromone detection. In adults, we previously described three putative PBP-encoding genes ( SlitPBP1, SlitPBP2, SlitPBP3 ) and four candidate PRs ( SlitPR6, SlitPR11, SlitPR13, SlitPR16 ), all of which are expressed in the antennae [15] . Using RT–PCR, we demonstrated that the three PBPs were also expressed in the larval antennae ( Fig. 5a ). By contrast, we were not able to amplify any of the four candidate PRs in the larval antennae cDNA, although ORco (OR coreceptor), which encodes an obligatory co-receptor of all ORs [16] , could be amplified ( Fig. 5a ). In view of these findings, we investigated the expression patterns of the three PBPs in the larvae antennae using whole-mount in situ hybridization. In the control experiments, no labelling was visible ( Fig. 5b ). The hybridizations using each PBP -labelled probe revealed a conserved expression pattern for the three PBPs , with two labelled spots clearly visible on segment II and one on segment III at the bases of the three olfactory sensilla ( Fig. 5b ). 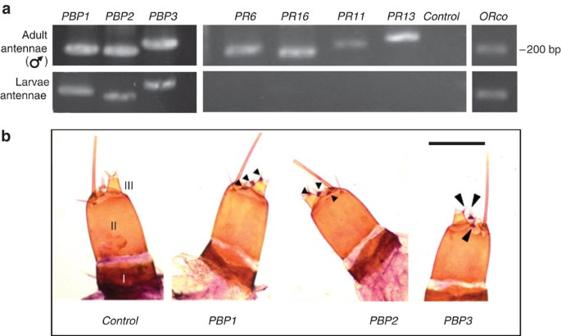Figure 5:PBPgene expression inS. littoralislarval antennae. (a) RT–PCR analyses of thePBP,ORcoandPRgene expression in the antennae of adult males and L3-L4 larvae. Control: water template. (b) Whole-mountin situhybridizations using dig-labelledPBP1,PBP2andPBP3antisense RNA probes (×400). Blue-labelled spots are visible at the bases of two sensilla of the antennal segment II and on one sensillum of segment III. Controls consisted of a mix of dig-labelled and unlabelled antisense RNA probes (ratio 1/100). Bar, 500 μm. Figure 5: PBP gene expression in S. littoralis larval antennae. ( a ) RT–PCR analyses of the PBP , ORco and PR gene expression in the antennae of adult males and L3-L4 larvae. Control: water template. ( b ) Whole-mount in situ hybridizations using dig-labelled PBP1 , PBP2 and PBP3 antisense RNA probes (×400). Blue-labelled spots are visible at the bases of two sensilla of the antennal segment II and on one sensillum of segment III. Controls consisted of a mix of dig-labelled and unlabelled antisense RNA probes (ratio 1/100). Bar, 500 μm. Full size image Taken together, these results demonstrate that the larval antennae express the three adult PBPs in the olfactory sensilla but that no PRs are expressed. Our behavioural and sensory data show that physiological doses of the sex PGEs attract caterpillars and activate their antennal ORNs. Both behavioural and electrophysiological responses showed characteristics that are typical for olfactory responses [7] , [17] . Wax-embedding the antennae completely suppressed this behaviour, suggesting that caterpillar palps are not involved in pheromone detection. As PGE may contain cues other than the sex pheromone, we then tested the synthetic main sex pheromone component that was proven to have behavioural and electrophysiological effects comparable to those of the gland extract. To investigate whether pheromone recognition is species specific or whether caterpillars would be able to respond to other moth pheromone molecules with different chain lengths, double-bond numbers or positions, we challenged caterpillars with a sex PGE from another noctuid, M. brassicae . This species was chosen because its sex pheromone is composed of a blend of acetate components [18] , but has chain lengths, double-bond numbers, and positions that are different from those of the S. littoralis pheromone. Interestingly, the M. brassicae pheromone blend did not elicit any behavioural response from the S. littoralis caterpillars, although it was detected by the antennae. These results suggest that S. littoralis caterpillars can clearly discriminate the pheromones of the two species. To our knowledge, only one study in the literature, which focused on B. mori , has used the sex pheromone in a behavioural test aimed at identifying attractants to caterpillars [7] . In contrast to our results, B. mori larvae showed no attraction to the species-specific sex pheromone. The behavioural setups used in the two studies may account for these differences; whereas Tanaka et al . [7] used closed boxes, we used a servosphere that made it possible to explore odorant-mediated anemotaxis under continuous air-flow in an open field. It has been demonstrated that odorant gradients form in closed spaces upon odorant loading and are stable for at least 15 min in, for example, a 96-well plate [19] . Long exposures, such as the 2-h exposure reported for B. mori larvae [7] , may thus lead to an uncontrolled gradient or to air saturation, thereby preventing the correct attraction. Because we demonstrated that caterpillars detect both the sex pheromone blend and Z9,E11-14:Ac through their antennae, we reasoned that they may use the same proteins as adults to recognize these stimuli, namely PBPs and PRs. We found that the three PBP-encoding genes previously identified in S. littoralis adult antennae are expressed in the caterpillar antennae. Furthermore, detailed expression studies revealed that all the three PBPs are expressed in the three olfactory sensilla carried by the antennae, including the sensillum from which we recorded a firing response to the pheromone stimulation. We did not detect the expression of any of the four candidate PR-encoding genes that we previously identified in the adults, which is in agreement with previous studies that have reported that PR genes are expressed exclusively in adults [7] , [10] , [11] . Thus, whereas the presence of PBPs makes the transport of adult sex pheromones possible in the olfactory sensilla of the larval antennae, the question arises as to whether the pheromone signal could be detected without the corresponding receptor. The four S. littoralis PR candidates studied here have been annotated as PRs based solely on a phylogenetic analysis [15] , and none have been functionally characterized. Therefore, it is possible that the S. littoralis PRs remain to be identified. Alternatively, caterpillars may use different receptors than adults to detect the same odorants. In B. mori , adults use an adult-specific PR to detect bombykol [7] , [20] , whereas larvae were shown to express a larva-specific receptor that responds to this compound [7] . Similarly, an endogenous OR sensitive to bombykol, which is different than the B. mori bombykol PR, has been discovered in the fruit fly Drosophila melanogaster [21] . However, the ecological significance of these observations is still unknown. The unexpected response of caterpillars to the sex pheromone raises the question of why these immature insects that do not care about finding a mate should be attracted to the female sexual signal. Contrary to the adult behaviour, in which only the males are attracted to the sex pheromone emitting females, our results show that larvae are attracted to the sex pheromone regardless of the sex of the forthcoming adult. Therefore, this signal is not used as a sex pheromone by larvae. One could argue that the late instar larvae start expressing the future adult genes required to detect the pheromone. However, both young and old larvae respond to this cue. S. littoralis larvae may use the pheromone signal to aggregate at a common site that could favour future mating or to enhance food intake. However, no aggregation behaviour has been reported for S. littoralis larvae. Very recently, the detection of food-derived odours has been shown to promote male courtship in D. melanogaster [22] . Similarly, it is possible that the detection of the sex pheromone promotes food search in caterpillars. In accordance with this latter hypothesis, in this study, the larvae were more attracted to a food source containing Z9,E11-14:Ac than to food that does not contain this sex pheromone component. Because plant odours are complex and variable and are composed of ubiquitous and specific chemicals, the recognition task is not easy for a caterpillar equipped with less than 80 ORNs and only a few ORs [1] , [7] , especially for a highly polyphagous species such as S. littoralis [23] . On the contrary, female antennae house a great number of ORNs tuned to plant volatiles [24] , which females use to find and more efficiently discriminate the future larval substrate when ovipositing. In this context, the sex pheromone emitted by calling females may act as a relevant cue for larvae to find appropriate hosts. Indeed, it is possible that females preferentially call for males in a host plant environment. During the calling process, the sex pheromone can adsorb to the leaf surface, as previously demonstrated in moths [25] . The female can then leave a crucial signal to the larvae. Alternatively, females may release traces of pheromone on appropriate leaves while ovipositing because the ovipositor and the pheromone gland are closely associated. Sex pheromones have been shown to enhance parasitism rates in egg parasitoids [26] , suggesting that sex pheromone traces are indeed present on eggs. Noticeably, neither newly hatched larvae of S. littoralis nor third instar larvae with prior experience of only a synthetic diet respond to odours from cotton leaves [27] . In this species, larval feeding has been shown to be influenced by previous feeding experience [28] . It has been proposed that the ability of these larvae to demonstrate a preference for an odour associated with a food source simplifies foraging [27] . Therefore, it is possible that newly hatched S. littoralis caterpillars experience the sex pheromone (either adsorbed on the leaves from calling females or deposited on the eggs) while eating their first leaf, a signal that they will further associate with the food source. Our study adds a new example of a multifunctional signal in the field of chemical ecology. Although sex pheromones are already known to act as kairomones for parasitoids, we suggest here a different role of pheromones in individuals of the same species according to their developmental stage. In the context of plant protection, this unexpected larval behaviour may provide new opportunities to manipulate the behaviour of herbivorous caterpillars, such as S. littoralis larvae. Insect rearing S. littoralis and M. brassicae were reared in the laboratory on a semi-artificial diet at 24 and 20 °C, respectively, at 60 to 70% relative humidity and under a 16:8 light:dark cycle. Larvae were kept in a separate room from the adults and had no contact with any sex pheromone source before the bioassays. Compounds and PGEs Hexanol (98% purity) and mineral oil were purchased from Aldrich (St Louis, MO, USA). Hexane (>98% purity) was purchased from Carlo-Erba. Z9,E11-14:Ac (( Z , E )-9,11-tetradecadienyl acetate, >97% purity) and Z11-16:Ac (( Z )-11-hexadecenyl acetate, >99% purity) were synthesized in the laboratory (courtesy of Martine Lettere). The pheromone glands of 2-day-old S. littoralis or M. brassicae females were dissected during their calling period and extracted with hexane (batches of 20 glands in 200 μl) for 1 h. All of the extracts were titered in sex pheromone by gas chromatography-mass spectrometry by determining the amount of their respective main components, namely Z9, E11-14:Ac ( S. littoralis ) and Z11-16:Ac ( M. brassicae ). Behavioural experiments All of the experiments were performed using 24 h-starved larvae. To study the age effect, two different groups of larvae at different developmental stages were used, namely 3–6-day-old larvae (first or second instar, L1-L2) on one side and 12–15-day-old larvae (third or fourth instar, L3-L4) on the other side. The larvae were put at the top of a TrackSphere locomotion compensator LC-300 system (Syntech, Hilversum, The Netherlands) in light conditions. The larvae were left for 30 s on the locomotion setup under a 36-cm s −1 humidified air-flow for adaptation before stimulation. Odour stimulation was then introduced into the air-flow for 3 min. At the end of the experiment, the larvae were separated and reared until pupation for sex determination. L3-L4 larvae were tested with hexane or mineral oil (solvent controls), hexanol (10, 100 and 1,000 ng diluted in mineral oil), pheromone extracts of S. littoralis (0.03, 0.3, 1 and 3 FE, in hexane), pheromone extracts of M. brassicae (1 FE) and synthetic Z9,E11-14:Ac (10 ng in hexane). In all of the experiments, hexane was allowed to evaporate before testing. As quantified by gas chromatography-mass spectrometry, 1 FE of PGEs contained 5 and 20 ng of S. littoralis and M. brassicae main pheromone components, respectively. The L1-L2 larvae were tested with hexane or pheromone extracts of S. littoralis (1 FE). All of the larvae were tested only once. The larval paths were recorded and analyzed by Syntech TrackSphere v3.1 software (Syntech, Hilversum, The Netherlands). The path lengths and mean vectors were calculated using custom R programs [29] . Each larva that walked at least 100 mm during the test, irrespective of the path direction, was defined as activated. An activated larva was considered as attracted to the stimulus when the angle of the mean vector of its path was included in the quadrant centered upwind along the air-flow axis ( Fig. 1a ). This allowed us to compute activation and attraction ratios; namely, the number of activated larvae/total number of larvae and the activated larvae in the source area/total number of activated larvae, respectively. The percentages of activation and attraction within an experiment were analyzed with logistic regression to evaluate stimulus, sex and larval stage effects. The tests were performed using Minitab v.12, (Minitab Inc., State College, PA, USA). To test the involvement of the antennae in the behavioural response, the antennae of some of the L3-L4 larvae were covered with wax 24 h before the experiment. Alternatively, for the sham controls, wax was put on the heads close to the antennae but not covering them. The choice test was performed in a closed glass Petri dish (14.5 cm diameter). One regular diet spot (1 g plus 10 μl hexane) and one diet plus pheromone spot (1 g regular diet plus 10 ng Z9,E11-14:Ac) were located at opposite ends along the diameter. Eight to ten L3-L4 larvae were placed in the middle of the dish, after the solvent evaporated. The dish area was divided into two parts delimited by arc circles centered on the food spots (radius 5.5 cm) ( Fig. 3a ). The numbers of larvae in each area were computed at 0, 2, 4, 6, 10, 14, 20 and 30 min. A control experiment with 1 g of regular diet on each spot was also performed. The choice indexes were calculated as follow: [(number of larvae diet + pheromone area )-(number of larvae diet area )] / total number of larvae in the test. The choice indexes were compared with 0 (no preference) using a Mood test with Minitab v.12. Electrophysiological recordings Recordings were performed on immobilized L3-L4 larvae. A silver electrode (0.5 mm o.d.) was inserted into the larval body up to the head and connected to the electrical ground. The single sensillum recordings were obtained by inserting a tungsten electrode at the base of one sensillum. The preparation was placed into a continuous stream of charcoal-filtered and humidified air (16 ml s −1 ) emanating from a 10-ml disposable syringe. A fast three-way solenoid valve (LFAA 1201618H, Lee Valve, USA) driven by a microcontroller (DL-05DD, Koyo Electronics, Japan) was used to drive a second air stream (1 ml s −1 ) for 0.5 s through a glass capillary (Ringcaps 50–100 μl, Hirschmann, Singeco, San Diego, CA, USA) positioned at 1 cm from the antenna. This capillary contained a filter paper (15 × 1.5 mm) previously loaded with the odorant diluted in hexane. For each recording session, the sensillum was stimulated with hexane (control), with either an increasing series of sex PGEs from either S. littoralis or M. brassicae (0.25 to 3 FE) or synthetic Z9,E11-14:Ac (1.25 to 15 ng). In all of the experiments, hexane was allowed to evaporate before testing. The ORN activities were recorded for 3 s, starting 1 s before the stimulus presentation. To prevent adaptation, the inter-stimulus interval was 2 min. Each stimulus was presented only once. Eight to twelve insects were tested for each stimulus. The electrical signals (action potentials of different sizes from several neurons) were recorded with an amplifier (AI 401×10 probe, Axon Instrument, USA) and filtered (CyberAmp 320, Axon Instrument, USA; AC amplification, 10–2800 Hz Bessel band-pass filter). The data were sampled at 10 kHz with a data acquisition card (16-bit A/D, DT9803; Data Translation, USA) under the control of a custom program, dbWave [30] . The response to each stimulus was computed as the difference between the numbers of action potentials occurring during the stimulation minus the number of action potentials recorded during the 0.5-s before the stimulation (typically approximately 150 spikes s −1 , Supplementary Fig. S3 ). The responses to the pheromone were compared with the responses to hexane using the Mann–Whitney test in Excel (Microsoft, USA). The dose effects were analyzed using linear regression (Minitab v.12). RNA extraction and PCR Total RNAs from the L3-L4 larvae antennae and palps were extracted using the Qiagen RNeasy microkit (Qiagen, Hilden, Germany). The total RNA from 2-day-old male adult antennae was extracted with TRIzol Reagent (Invitrogen, Carlsbad, USA). The corresponding cDNAs were synthesized using the Advantage RT-for-PCR Kit (Clontech, Mountain View, USA). PCRs were performed for 35 cycles using specific primer pairs designed for each selected S. littoralis gene and Titanium Taq DNA polymerase (Clontech). The following primers were used: PBP1 forward primer: 5′-ATGGCGAAGAAGTTGGACCTC-3′, PBP1 reverse primer: 5′-CTCGTGGATCTTAGTGCGGAAG-3′; PBP2 forward primer: 5′-TTCTGGAAGGAAGGCTACGA-3′, PBP2 reverse primer: 5′-CAGGGTCTTCATGCAAGGAT-3′; PBP3 forward primer: 5′-GATGGATCGCGTAACGTCTT-3′, PBP3 reverse primer: 5′-CTCATGCTTGCATTCTTCCA-3′. Gene-specific primers for SlitrpL8 (used as an endogenous control), ORco and SlitPRs have previously been described [15] , [31] . The amplification products were loaded on 2% agarose gels and visualized using ethidium bromide. In situ hybridization Antennae from the L3-L4 larvae were fixed overnight in 4% paraformaldehyde. Digoxigenin-labelled and unlabelled RNA antisense probes (~400 bp in length) of S. littoralis PBP1 , PBP2 and PBP3 genes were transcribed in vitro from the PCR fragments using T7 RNA polymerases (Promega, Madison, WI, USA). The hybridizations were performed on whole-mount antennae as previously described [32] . The control experiments consisted of hybridization with a mix (1/100) of dig-labelled and unlabelled antisense probes. How to cite this article: Poivet, E. et al . The use of the sex pheromone as an evolutionary solution to food source selection in caterpillars. Nat. Comm. 3:1047 doi: 10.1038/ncomms2050 (2012).